A brain-wide functional map of the serotonergic responses to
acute stress and fluoxetine Central serotonin (5-HT) orchestrates myriad cognitive processes and
lies at the core of many stress-related psychiatric illnesses. However, the basic
relationship between its brain-wide axonal projections and functional dynamics is
not known. Here we combine optogenetics and fMRI to produce a brain-wide 5-HT evoked
functional map. We find that DRN photostimulation leads to an increase in the
hemodynamic response in the DRN itself, while projection areas predominately exhibit
a reduction of cerebral blood volume mirrored by suppression of cortical delta
oscillations. We find that the regional distribution of post-synaptically expressed
5-HT receptors better correlates with DRN 5-HT functional connectivity than
anatomical projections. Our work suggests that neuroarchitecture is not the primary
determinant of function for the DRN 5-HT. With respect to two 5-HT elevating
stimuli, we find that acute stress leads to circuit-wide blunting of the DRN output,
while the SSRI fluoxetine noticeably enhances DRN functional connectivity. These
data provide fundamental insight into the brain-wide functional dynamics of the 5-HT
projection system. The central nervous system (CNS)’s expansive serotonergic (5-HT) circuit
is amongst the most versatile and important neurotransmitter systems for emotional
and cognitive processing. Primarily originating within the phylogenetically ancient
dorsal raphe nucleus (DRN), a small brainstem nuclei that projects promiscuously
throughout the brain, the CNS 5-HT circuit influences mood, memory, circadian
rhythm, feeding, feeling of reward and stress coping, and is strongly implicated in
the aetiology and treatment of many prevalent neurological disorders, especially
those related to stress [1] , [2] , [3] , [4] . However, much remains
unknown about its basic character, particularly with respect to its functional
connectivity. For example, are the neural correlates of hemodynamic responses from
5-HT signalling the same as those for glutamatergic signalling? Does the anatomical
architecture of the 5-HT circuit correlate with its functional connectivity? How do
separate stimuli that lead to elevated synaptic 5-HT, e.g. selective serotonin
reuptake inhibitor (SSRI) and acute stress, affect the elicited circuits? To address these outstanding questions, we used optogenetic combined
with functional magnetic resonance imaging (ofMRI) [5] to establish a whole-brain
visualisation of the central 5-HT functional circuit in the live mouse. We find the
functional map to be indicative of bidirectional circuit regulation, and its
functional connectivity to better match regional expression of certain 5-HT receptor
subtypes than 5-HT neuron projection density. In addition, we find that delta
oscillations, more so than gamma oscillations or multi-unit activity (MUA), best
mirror hemodynamic changes associated with optogenetically evoked 5-HT release
across the cortex. When examining the circuit following either acute stress or
administration of fluoxetine, we observe opposite effects on DRN 5-HT functional
connectivity, providing an elegant explanation at the circuit level for the
behavioural divergence of these stimuli. Our observations underscore the power of
ofMRI for characterizing large brain networks originating from subcortical nuclei,
as well for analysing effects of acute stimuli on neuromodulatory systems. A whole-brain functional map of the DRN 5-HT circuit To identify and control the activity of midbrain neurons expressing Pet-1 , a gene critical for 5-HT neuron
development and function, we injected a Cre-inducible viral construct encoding
Channelrhodopsin-2 fused to enhanced yellow fluorescent protein (ChR2-eYFP) into
the DRN of ePet-Cre +/− mice (Fig. 1a ). In these ePet DRN ::ChR2-eYFP mice, 96.1 ± 0.8% (mean ± 1 standard deviation) of ChR2-expressing DRN neurons
co-stained for 5-HT, demonstrating highly specific targeting of serotonergic
neurons, with 75.4 ± 5.4% of 5-HT-immunopositive neurons coexpressing ChR2-eYFP
( n = 3 mice; Fig. 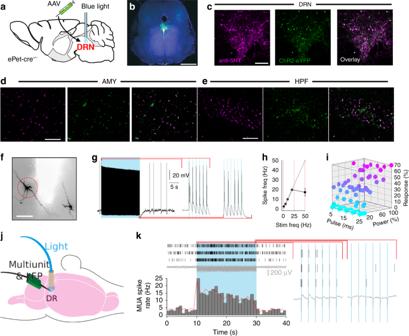Fig. 1 Optogenetic targeting of DRN 5-HT neurons.aInfusion of AAV harbouring
cre-dependent ChR2-eYFP into the DRN ofePet-cre+/−mice, followed by
implantation of a MRI-friendly optic fibre used to deliver blue
light.bWhole midbrain slice
with Ch2R in green. DAPI (blue) identify all cell nuclei. Scale
bar indicates 2.5 mm.c–eCo-immunofluorescence with anti-5-HT (purple) and ChR2-eYFP
(green) in the (c) DRN,
(d) amygdala (AMY) and
(e) hippocampus (HPF).
Scale bars indicate 500, 100 and 50 µm, respectively.fBiocytin-filled neurons of the DRN
used for in vitro whole-cell patch electrophysiology. Red dashed
circle indicates recorded neuron. Scale bar indicates 200 µm.gResponse of neuron
circled in (f) to all but one
pulse of a blue light train.hFrequency response curve from midbrain slices. Linearity stable
to 20 Hz.iStrength of
response expressed in maximum number of spikes per pulse during
20 Hz photostimulation, as a function of pulse width and laser
power.jSchematic of the
experimental set-up for paired MUA and LFP recordings in the DRN
during photostimulation.kRaster plots of MUA activity in three neighbouring channels
(top), LFP (middle) and mean spike histogram (bottom), revealing
activation of the DRN 5-HT network during a blue light train
(20 Hz, 5 ms pulse width). Expanded to the right are the MUA and
LFP for the first and last 6 pulses in the train 1b, c , Supplementary Figure 1 ). While no ChR2-eYFP-positive cell bodies
were found outside the DRN (Fig. 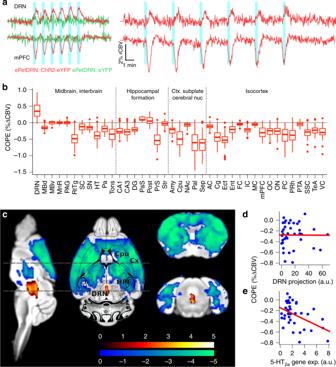Fig. 2 A whole-brain functional map of the DRN 5-HT circuit.aCBV traces from the DRN
and medial prefrontal cortex (mPFC) during block stimulation
with blue light (20 Hz, 5 ms pulse width, 6 × 20 s trains)
during the short (ePetDRN::ChR2-eYFP,n= 10,ePetDRN::eYFP,n= 4) and long (ePetDRN::ChR2-eYFP,n= 7) fMRI protocols.bContrast of parameter estimates (COPEs)
extracted across 39 ROIs fromePetDRN::ChR2-eYFPusing the short protocol (n= 10). They denote the relative
response amplitude across the brain. Bound of box and centre
line represent 25th, 50th, 75th percentiles, whiskers represent
1.5*inter-quartile range.cSecond level voxel-wise analysis ofePetDRN::ChR2-eYFP(n= 10) againstePetDRN::eYFP(n= 4). Cx cortex, Cpu caudate-putamen, HPF
hippocampal formation, DRN dorsal raphe nucleus. Colour
scale =t-statistic
(non-parametric test,p≤ 0.05, cluster corrected).d,eCOPEs
extracted from 38 ROIs compared withdDRN projection field estimated with viral
tracer ande5-HT2Agene expression estimated with
in-situ hybridization, both obtained from AIBS
database 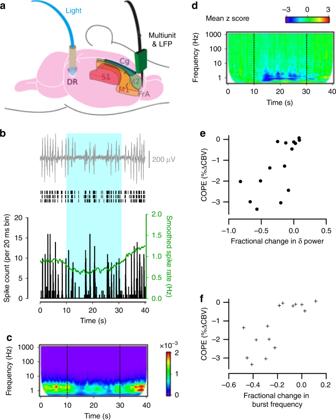Fig. 3 Photoactivation of DRN 5-HT neurons dampens MUA and LFP
power in cortical projection areas.aSchematic of the experimental set-up for
paired MUA and LFP recordings in the DRN and projection areas
during photostimulation.bCortical LFP (top), raster plots (middle) of spikes recorded on
3 neighbouring channels and spike time histogram (bottom),
reveal reduction in the frequency of cortical network bursts and
MUA during optogenetic activation of DRN 5-HT neurons.cWavelet amplitude spectrum of the
cortical LFP averaged over 6 stimulation trials for the
experiment shown in (b) (warmer
colours indicate higher power). Dashed lines indicate onset and
end of photostimulation.dZ
transform of the wavelet amplitude spectrum averaged across
recording sites of mice with robust CBV response to
photostimulation, showing a consistent reduction in the
amplitude of low-frequency LFP components (8 recording sites
from 3 mice).e,fCOPEs from various cortical regions
correlate strongly with fractional changes in both theddelta power (Pearsonr= 0.69;p= 0.004) andeburst frequency (Pearsonr= 0.78;p= 0.0006) recorded in 15 recording sites from
7 mice 1b, c ),
axons co-expressing ChR2-eYFP and 5-HT were found terminating in the neocortex
(Supplementary Figure 2 ), thalamus
(Supplementary Figure 3 ), amygdala
(Fig. 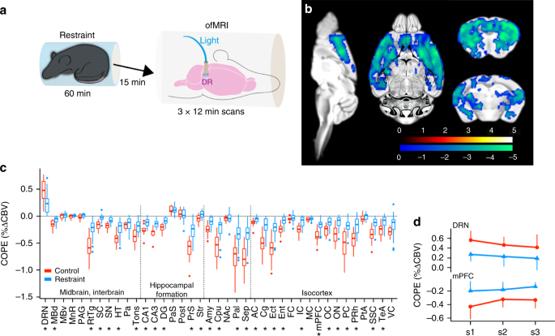Fig. 4 Acute stress occludes photoactivation of the DRN 5-HT
circuit.aExperiment
schematic.bSecond level
analysis comparing restraint (n= 7) to control (n= 4) condition indicate a decrease in negative
response amplitude in the restraint group relative to control
across the brain. Colour scale =t-statistic (non-parametric test,p≤ 0.05, cluster corrected), blue
indicating significance for restraint > control
comparison; see Supplementary Figure13for all brain slices.cCOPEs comparing restraint (blue)
and control (red) indicate reduced response amplitudes in the
majority of responding ROIs, including DRN (*p< 0.05, FDR corrected).
Bound of box and centre line represent 25th, 50th, 75th
percentiles, whiskers represent 1.5*inter-quartile range.dThe blunted response to
photoactivation following acute stress persists across the three
consecutive scans of each session. Error bars indicate ±1
standard deviation 1d ; Supplementary
Figure 4 ), dorsal hippocampus
(Fig. 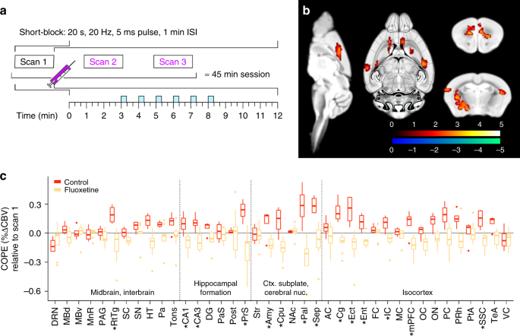Fig. 5 Circuit regulation of DRN 5-HT functional connectivity
by fluoxetine.aExperiment
schematic.bSecond level
analysis comparing fluoxetine (n= 9) to control (n= 4) condition indicate an increase in
negative response amplitude in scan 2 and 3 relative to scan 1
in the prefrontal, cingulate and peri-hippocampal cortex, as
well as amygdala and parts of the striatum, in the fluoxetine
group. Colour scale =t-statistic (non-parametric test,p≤ 0.05, cluster corrected),
red-yellow colour bar indicating significance for
fluoxetine < control comparison; see Supplementary
Figure15for all
brain slices.cCOPEs comparing
fluoxetine (yellow) and control (red) confirm an augmentation of
the decreased response amplitudes in CBV within regions
highlighted by the voxel-wise analysis (*p< 0.05, FDR corrected). Bound of box
and centre line represent 25th, 50th, 75th percentiles, whiskers
represent 1.5*inter-quartile range 1e ; Supplementary
Figure 5 ) and striatum
(Supplementary Figure 6 ). Consistent
with earlier reports, these data highlight the structural substrate by which
midbrain-derived serotonin neurons could modulate nearby and distant brain
regions [2] . To ascertain the efficacy of the opsin, we
performed electrical recordings during blue light illumination in vitro and
found neurons stimulated with a 5 ms pulse remained faithful to a 20 s, 20 Hz
stimulus train, even in the presence of anaesthetic (Fig. 1f–i , Supplementary Figure 7 ). This paradigm was found to maximise spiking
recorded within the DRN while minimizing duty cycle. Block lengths was optimized
for ofMRI detection to correspond to 10 volumes in our acquisitions. Importantly, the paradigm was selected to induce contrasting level of activity
relative to baseline and may not reflect DRN physiological activity. Fig. 1 Optogenetic targeting of DRN 5-HT neurons. a Infusion of AAV harbouring
cre-dependent ChR2-eYFP into the DRN of ePet-cre +/− mice, followed by
implantation of a MRI-friendly optic fibre used to deliver blue
light. b Whole midbrain slice
with Ch2R in green. DAPI (blue) identify all cell nuclei. Scale
bar indicates 2.5 mm. c – e Co-immunofluorescence with anti-5-HT (purple) and ChR2-eYFP
(green) in the ( c ) DRN,
( d ) amygdala (AMY) and
( e ) hippocampus (HPF). Scale bars indicate 500, 100 and 50 µm, respectively. f Biocytin-filled neurons of the DRN
used for in vitro whole-cell patch electrophysiology. Red dashed
circle indicates recorded neuron. Scale bar indicates 200 µm. g Response of neuron
circled in ( f ) to all but one
pulse of a blue light train. h Frequency response curve from midbrain slices. Linearity stable
to 20 Hz. i Strength of
response expressed in maximum number of spikes per pulse during
20 Hz photostimulation, as a function of pulse width and laser
power. j Schematic of the
experimental set-up for paired MUA and LFP recordings in the DRN
during photostimulation. k Raster plots of MUA activity in three neighbouring channels
(top), LFP (middle) and mean spike histogram (bottom), revealing
activation of the DRN 5-HT network during a blue light train
(20 Hz, 5 ms pulse width). Expanded to the right are the MUA and
LFP for the first and last 6 pulses in the train Full size image To determine whether the activity of serotonergic neurons affect
target structure cell activity, we combined in vivo multiunit recordings with
photostimulation in 5 ePet DRN ::ChR2-eYFP mice and 2 WT DRN ::ChR2-eYFP control mice anaesthetised using an anaesthesia
regime optimised for small animal functional magnetic resonance imaging (fMRI)
(0.5% isoflurane + 0.2 mg/kg/h s.c. medetomidine) [6] . In ePet DRN ::ChR2-eYFP mice, the firing rate of DRN neurons increased in
response to blue light stimulation (Fig. 1j,
k ). Putative unit waveform subtypes did not exhibit any
significant differences in the probability of spiking in response to single
low-frequency light pulses (Kruskal–Wallis = 0.76, p = 0.68) or 20 Hz pulse trains (Kruskal–Wallis = 1.51, p = 0.47), indicating that
photostimulation recruited a range of DRN 5-HT neuron subtypes with differing
intrinsic electrophysiological properties (Supplementary Figure 8 ). We did however note that putative units in
the intact DRN never fired at or close to 20 Hz in vivo (Supplementary
Figure 8c ), despite the fact that
patched 5-HT cells in acute midbrain slices remained faithful to the train up to
20 Hz (Fig. 1h ). While over-clustering
could lead to an underestimation of the individual unit firing rates, even the
MUA recorded at the most active electrodes in the DRN in vivo did not achieve
rates of 20 Hz during light train stimulation. This profound contrast between in
vitro and in vivo fidelity at the single neuron level may be the result of local
or distal feedback regulation within the intact DRN 5-HT circuit. The functional
role of the different 5-HT neuron subtypes identified, in particular how they
elicit different circuit elements, remains to be elucidated. To measure brain-wide responses to DRN serotonergic photoactivation,
we recorded changes in cerebral blood volume (CBV) during optogenetic
stimulation (ofMRI) using a block protocol consisting of 6 × 20 s, 20 Hz
stimulus trains delivered either every 1 min or every 3 min (Fig. 2a ). The acquired images presented minimal motion
(mean frame-wise displacement 0.021 ± 0.008 mm) and geometric distortions,
despite the implant (Supplementary Figure 9a–c ). The method was preferred over blood oxygenation level
dependent contrast (BOLD) due to enhanced detection power, suppression of large
vessel signal and reduced susceptibility artefact (Supplementary
Figure 9a, f,
g ) [7] . Importantly, CBV contrast leads to a
seven-fold increase in response amplitude relative to that recorded with BOLD. In both stimulus paradigms, we found that CBV increased within the DRN during
illumination, while projection areas including the medial prefrontal cortex
predominately exhibited a tightly stimulus-locked CBV decrease, followed by an
immediate return to baseline and rebound overshoot. Interestingly, the amplitude
of the response decreased over the course of the six stimulation blocks in the
projection areas, from 2.6% to 1.7%, but not in the DRN, suggesting an
adaptation to enhanced 5-HT release within the DRN or projection areas. The
shorter inter-block protocol was adopted to allow the acquisition of several
scans within a single scan session. The CBV response was fitted with a general
linear model (GLM) to facilitate unbiased voxel-wise comparisons between
conditions across the entire brain. Contrast of parameter estimates (COPEs),
representing the regional response amplitude, were estimated from every voxel
using a gamma function model (Fig. 2b ,
Supplementary Figure 9d ). A
second-level comparison across the whole brain between ePet DRN ::ChR2-eYFP ( n = 10) and ePet DRN ::eYFP ( n = 4) revealed the extent of the
elicited response, including a positive response confined within the DRN, and a
negative CBV response distributed among the hippocampal formation, cortical
subplate and striatum, and isocortex (Fig. 2d ). Illumination in the absence of ChR2 produced no
significant response, ruling out the possibility of light-induced heating
artefacts (Fig. 2a , Supplementary
Figure 9e ). Interestingly, there
was spatial overlap regarding the distal CBV response elicited with optogenetic
stimulation with that evoked with chemogenetic stimulation of the 5-HT DRN
neurons [8] , though the directionality of the response
was opposed, and only optogenetically-induced responses matched the
directionality of acute pharmacological stimulation of the DRN with a
SSRI [8] , [9] . This severe discrepancy between two recently
emerged stimulation methods, often discussed interchangeably in neuroscience
research, exemplifies the potential extreme non-linear effects induced with
acute and selective circuit manipulations [10] . Indeed, the activity
evoked departs from basal physiological 5-HT firing patterns, which may explain
this discrepancy. This highlights the relevance of intact whole-circuit
visualisation in support of behavioural observations or other modalities. Fig. 2 A whole-brain functional map of the DRN 5-HT circuit. a CBV traces from the DRN
and medial prefrontal cortex (mPFC) during block stimulation
with blue light (20 Hz, 5 ms pulse width, 6 × 20 s trains)
during the short ( ePet DRN ::ChR2-eYFP , n = 10, ePet DRN ::eYFP , n = 4) and long ( ePet DRN ::ChR2-eYFP , n = 7) fMRI protocols. b Contrast of parameter estimates (COPEs)
extracted across 39 ROIs from ePet DRN ::ChR2-eYFP using the short protocol ( n = 10). They denote the relative
response amplitude across the brain. Bound of box and centre
line represent 25th, 50th, 75th percentiles, whiskers represent
1.5*inter-quartile range. c Second level voxel-wise analysis of ePet DRN ::ChR2-eYFP ( n = 10) against ePet DRN ::eYFP ( n = 4). Cx cortex, Cpu caudate-putamen, HPF
hippocampal formation, DRN dorsal raphe nucleus. Colour
scale = t -statistic
(non-parametric test, p ≤ 0.05, cluster corrected). d , e COPEs
extracted from 38 ROIs compared with d DRN projection field estimated with viral
tracer and e 5-HT 2A gene expression estimated with
in-situ hybridization, both obtained from AIBS
database Full size image DRN photoactivation suppresses cortical neuronal activity For fMRI responses in the monkey visual cortex elicited by rotating
polar-transformed chequerboard patterns, a cognitive process mediated by
glutamatergic and GABAergic signalling amongst networks of pyramidal neurons and
interneurons, local field potentials (LFPs) were found to better estimate the
BOLD response compared to MUA [11] . This finding suggested that fMRI
hemodynamic signals reflect the input to, and intracortical processing within, a
specific area rather than its spiking output [11] . However, it remains
unclear whether this observation can be generalised to other forms of neuronal
communication such as 5-HT mediated signalling. We therefore performed
intracranial recordings from a variety of cortical regions and compared LFP and
spiking behaviour with the hemodynamic response to transient photoactivation of
DRN 5-HT neurons (Fig. 3a ). Fig. 3 Photoactivation of DRN 5-HT neurons dampens MUA and LFP
power in cortical projection areas. a Schematic of the experimental set-up for
paired MUA and LFP recordings in the DRN and projection areas
during photostimulation. b Cortical LFP (top), raster plots (middle) of spikes recorded on
3 neighbouring channels and spike time histogram (bottom),
reveal reduction in the frequency of cortical network bursts and
MUA during optogenetic activation of DRN 5-HT neurons. c Wavelet amplitude spectrum of the
cortical LFP averaged over 6 stimulation trials for the
experiment shown in ( b ) (warmer
colours indicate higher power). Dashed lines indicate onset and
end of photostimulation. d Z
transform of the wavelet amplitude spectrum averaged across
recording sites of mice with robust CBV response to
photostimulation, showing a consistent reduction in the
amplitude of low-frequency LFP components (8 recording sites
from 3 mice). e , f COPEs from various cortical regions
correlate strongly with fractional changes in both the d delta power (Pearson r = 0.69; p = 0.004) and e burst frequency (Pearson r = 0.78; p = 0.0006) recorded in 15 recording sites from
7 mice Full size image Similarly to the glutamatergic response to a behavioural
stimulus [11] , the 5-HT response to photoactivation
represents synaptic signal integration. Specifically, synchronous with
photoactivation of DRN 5-HT neurons, cells in the frontal, somatosensory, motor
and anterior cingulate cortex exhibited stimulus-evoked decreases in both MUA
and LFP power that rapidly returned to baseline upon stimulus termination
(Fig. 3b ). Wavelet analysis revealed
that delta bands were most affected, gradually declining in power upon
optogenetically-triggered 5-HT release in the cortex and returning to baseline
upon termination of the stimulus train (Fig. 3c,
d ). Changes to LFP power occurred following a post-stimulus
delay of about 5 s. We also observed that the fractional cortical delta power
(Fig. 3e ) and the fractional change
in burst frequency (Fig. 3f ) were both
inversely correlated with between-subject and regional variance in response
amplitude measured in the same group of animals during ofMRI. The convolved
LFP-derived band power correlated markedly with the CBV response evoked by 5-HT
release ( r delta = 0.75 ± 0.16, r gamma = 0.24 ± 0.6, Supplementary
Figure 10 ), while no discernible
correlations could be established between convolved MUA signal and CBV
( r MUA = -0.1 ± 0.34) for animal- and region of
interest (ROI)-matched recordings. ofMRI response is independent of projection density We next investigated cellular and molecular factors determining
functional connectivity of the DRN 5-HT circuit by comparing the whole-brain
DRN/5-HT hemodynamic maps derived from ofMRI with the DRN/5-HT neuron projection
density maps from the Allen Institute for Brain Science (AIBS). Prior to this
comparison, we removed white matter structures from the projection maps to
ensure that our analysis focused on 5-HT terminals rather than fibre tracts
(Supplementary Figure 11 ). Surprisingly, we did not find significant correlations (Fig. 2d , Supplementary Figure 12a ) indicating that the anatomical
architecture of the central 5-HT circuitry as such does not determine the
functional consequences of its activation. These results are consistent with the
finding that functional connectivity originating from photoactivated dopamine
neurons of the ventral tegmental area (VTA) does not correlate well with VTA
dopaminergic neuron projection density [12] , but are in stark
contrast to recent resting-state fMRI observations that indicate intracortical
functional connectivity relationships at a macroscopic level correlate with
intracortical structural connectivity [13] , [14] , [15] . We therefore examined another possible determinant for
regional-variance of hemodynamic responses elicited by DRN 5-HT
photostimulation, namely the specific expression patterns of 5-HT receptors. The
5-HT receptor family is comprised of both metabotropic and ionotropic sub-types
that can be either excitatory or inhibitory, depending on downstream signalling
cascades and cellular localisation [1] , and may strongly influence the net
effect of 5-HT release on functional connectivity. We explored this possibility
using a series of additional brain-wide voxel correlation maps from the best
available 5-HT receptor subtype expression data currently available from the
AIBS. Of the 14 5-HT receptor subtypes listed in the database, we judged 5
expression maps to be sufficiently robust for our analysis (Supplementary
Figure 11 ); the remaining AIBS
maps either containing strong artefacts or no signal. Significant correlations
emerged between the patterns of 5-HT 1F ,
5-HT 2A and 5-HT 2C receptor
density and the hemodynamic response, while distribution of
5-HT 1A and 5-HT 1B receptors
did not match the ofMRI response pattern, similar to the comparison with DRN
5-HT projections (Fig. 2e , Supplementary
Figure 12b–f ). Since we were
unable to assess all 5-HT receptor subtypes, we cannot conclude whether these
first three receptor subtypes determine functional connectivity of the DRN 5-HT
circuit; nevertheless, 5-HT 1F/2A/2C explain 52.6%, 21.2%
and 30.8% of the variance in the hemodynamic response elicited by DRN 5-HT
photostimulation, respectively. Interestingly, 5-HT 1A and
5-HT 1B receptors are autoreceptors expressed either
somatodendritically on 5-HT neurons of the DRN or presynaptically within axon
terminals of DRN 5-HT neurons [16] , [17] , while 5-HT 1F ,
5-HT 2A and 5-HT 2C receptors
are all expressed post-synaptically [18] , [19] . We therefore conclude that post-synaptic
receptor density, compared to neuroarchitecture, is the rather surprising
dominant factor underlying DRN 5-HT functional connectivity following our
photoactivation protocol. All remaining variance is likely governed by indirect
poly-synaptic connections, an expected contribution given other recent fMRI
findings [15] . This finding may hold for other
neuromodulatory systems including dopamine and neuropeptides as well, for which
projection density can be surprisingly sparse in regions that exhibit high
levels of receptor expression. Ultimately, the emerging data depict a potential
level of macro plasticity in neuromodulatory circuits that could not be attained
if neuroarchitecture dominated neuroconnectivitiy, as has previously been
assumed [20] . Acute stress occludes the ofMRI response The DRN represents an important element of the acute stress
response [21] , [22] , exemplified by activation of 5-HT neurons
and an increase in the synaptic availability of 5-HT throughout much of the
brain following forced restraint [23] , [24] . To determine how functional circuit changes
might be affected by acute stress, we subjected 7 ePet DRN ::ChR2-eYFP mice to a brief immobilisation period immediately prior to ofMRI and compared
the results to 4 ePet DRN ::ChR2-eYFP stress-free controls (Fig. 4a ). We found a marked reduction in the hemodynamic response
to DRN 5-HT photoactivation in acutely-stressed animals versus controls
(Fig. 4b, c ; Supplementary Figure 13 ). Moreover, this effect
persisted throughout three successive ofMRI scans (Fig. 4d ), indicating that the consequences for DRN
5-HT function elicited by acute stress persisted throughout the duration of the
experiment. Fig. 4 Acute stress occludes photoactivation of the DRN 5-HT
circuit. a Experiment
schematic. b Second level
analysis comparing restraint ( n = 7) to control ( n = 4) condition indicate a decrease in negative
response amplitude in the restraint group relative to control
across the brain. Colour scale = t -statistic (non-parametric test, p ≤ 0.05, cluster corrected), blue
indicating significance for restraint > control
comparison; see Supplementary Figure 13 for all brain slices. c COPEs comparing restraint (blue)
and control (red) indicate reduced response amplitudes in the
majority of responding ROIs, including DRN (* p < 0.05, FDR corrected). Bound of box and centre line represent 25th, 50th, 75th
percentiles, whiskers represent 1.5*inter-quartile range. d The blunted response to
photoactivation following acute stress persists across the three
consecutive scans of each session. Error bars indicate ±1
standard deviation Full size image Since the hemodynamic responses were blunted by acute stress within
DRN projection areas as well as the DRN itself, we normalised the COPEs of
projection areas to the COPE of the DRN to determine whether the functional
connectivity of the DRN 5-HT circuit was affected. No statistical difference
between acutely restrained animals and controls was apparent (Supplementary
Figure 14 ), indicating that
following acute stress, functional connectivity per se is actually not
affected. We presume the global blunting effects of stress on photoactivation
represent a ceiling effect since stress can lead to DRN sensitisation
accompanied by sustained increases in 5-HT release for up to
24 h [25] , [26] , [27] . Such a scenario would
produce less room for further inhibition, attenuating the hemodynamic response
to DRN 5-HT neuron photoactivation, which is what we observed here. The change
in response amplitude following restraint highlights the potential of ofMRI for
investigating neurological implications of salient life experiences. The
amplitude of photoactivation-elicited responses may serve as a measurable and
objective proxy for stress, enabling detailed examination of procedures that
might support stress resilience, such as anxiolytic agents and behavioural
enrichment. Circuit regulation of DRN 5-HT connectivity by fluoxetine As the primary source of 5-HT for the CNS, the DRN is presumed
critical for SSRIs mode of action. However, the mechanism underlying the effect
of SSRIs on the intact DRN 5-HT circuit remains unclear beyond the knowledge
that fluoxetine, like acute stress, elevates synaptic availability of
5-HT [28] . We therefore used ofMRI to study SSRIs by
administering a pharmacologically relevant dose [29] of fluoxetine via tail
vein infusion during ofMRI in 9 ePet DRN ::ChR2-eYFP mice and compared the results to 4 ePet DRN ::ChR2-eYFP non-injected controls (Fig. 5a ). Fluoxetine administration elicited greater response amplitude in the prefrontal
and cingulate cortex, as well as amygdala and striatum (Fig. 5b, c , Supplementary Figure 15 ). The ability to monitor animals
non-invasively with ofMRI is thus expected to reveal the circuit re-organisation
taking place longitudinally and shed light on currently obscure mechanisms of
anti-depressant action. Fig. 5 Circuit regulation of DRN 5-HT functional connectivity
by fluoxetine. a Experiment
schematic. b Second level
analysis comparing fluoxetine ( n = 9) to control ( n = 4) condition indicate an increase in
negative response amplitude in scan 2 and 3 relative to scan 1
in the prefrontal, cingulate and peri-hippocampal cortex, as
well as amygdala and parts of the striatum, in the fluoxetine
group. Colour scale = t -statistic (non-parametric test, p ≤ 0.05, cluster corrected),
red-yellow colour bar indicating significance for
fluoxetine < control comparison; see Supplementary
Figure 15 for all
brain slices. c COPEs comparing
fluoxetine (yellow) and control (red) confirm an augmentation of
the decreased response amplitudes in CBV within regions
highlighted by the voxel-wise analysis (* p < 0.05, FDR corrected). Bound of box
and centre line represent 25th, 50th, 75th percentiles, whiskers
represent 1.5*inter-quartile range Full size image The 5-HT system constitutes the most diverse signalling network of the
CNS and major physiological elements of its circuit characteristics remain unclear. Here we demonstrate the possibility to visualise the whole circuit in the intact
mammalian brain in conjunction with psychiatric-relevant stimuli. Several surprising
findings emerged from this analysis. First, we observe that photostimulation of the
DRN within ePet DRN ::ChR2-eYFP mice recruits a variety of 5-HT neuronal subtypes
distinguished by their waveforms. Second, this stimulation leads to an increase in
CBV within the DRN that coincides with decreases in CBV throughout much of the
brain, demonstrating that despite the expression of excitatory and inhibitory 5-HT
receptors, the net effect of 5-HT release in most areas is inhibitory. Third, the
hemodynamic response to photostimulation correlates with LFP delta oscillations and,
like glutamatergic-induced hemodynamic responses, likely corresponds to synaptic
integration rather than neuronal spiking. Fourth, functional connectivity of the DRN
5-HT network is rather remarkably uncoupled from its underlying neuroanatomical
architecture, and instead primarily governed by the far more plastic regional
differences in the expression profiles of post-synaptically expressed 5-HT
receptors. Fifth, acute stress shunts further activation of the DRN 5-HT circuit
without affecting absolute functional connectivity. Sixth, fluoxetine exerts the
opposite effect as acute stress by enhancing DRN 5-HT-induced suppression of brain
activity within restricted regions of the central 5-HT circuit. These results help understand basic principles of the DRN 5-HT circuit,
providing novel insights on the neural correlates underlying the hemodynamic
responses that follow DRN 5-HT neuron activation. The widespread inhibition observed
here contrasts with the subtle behaviour response mediated with 5-HT DRN
photostimulation, e.g. inhibition of spontaneous locomotor
activity [30] , inhibition of somatosensory
activity [31] , despite comparable paradigms. This apparent
discrepancy between visualized neuronal activity and behavioural outcome should be
explored in greater depth. For instance, ofMRI would provide a crucial tool to
explain behavioural variability in a population of animals. Additionally, these
results provide a potential neurophysiological explanation for the divergent
outcomes triggered by acute stress and acute fluoxetine administration, despite the
fact that both of these acute stimuli increase 5-HT synaptic availability. The most
important discovery however may be that post-synaptic receptor expression density,
and not DRN 5-HT neuroarchitecture, is the primary determinant of functional
connectivity within the central 5-HT system. Our study therefore highlights the
existence of a far more extended functional connectome relative to what structural
connectivity of the DRN alone would indicate. Experimental subjects All experiments and manipulations conformed to the guidelines set
by the Animal Care Commission of Switzerland and were covered under the
authority of animal permit ZH150/11 given to I.M.M. and ZH263/14 belonging to
B.J.S. and in accordance with the UK Animals (Scientific Procedures) Act 1986. All possible measures were taken to ensure minimal pain and discomfort. B6.Cg-Tg(Fev-cre)1Esd/J (ePet-cre mice;
RRID:IMSR_JAX:012712) males and females, 8–16 weeks of age, were used in this
study. ePet-cre Genotyping was complete using
forward primer AAAATTTGCCTGCATTACCG, reverse primer ATTCTCCCACCGTCACG and an
annealing temperature of 57 °C. Histology Fluorescent imaging: Animals were anesthetized with a lethal
cocktail of ketamine (120–150 mg kg −1 ) and
medetomidine (0.5–1.0 mg kg −1 ) administered i.p. and
then perfused with 10–15 ml ice-cold PBS followed by 10–15 ml ice-cold 4%
paraformaldehyde (PFA) in phosphate buffered saline (PBS). The whole brain was
then removed and stored in 4% PFA in PBS at 4 °C for at least 24 h. Brains were
sectioned on a vibratome (Leica, Germany), permeabilized with 0.1% Triton-X in
PBS for 10 min, processed according to target of interest (Supplementary
Table 1 ) and mounted in
VectaShield medium (Vector Laboratories, CA, USA) according to manufacturer
instructions. Fluorescence was captured using a Leica DFC365FX camera mounted on
a Leica M165F6 wide-field fluorescent stereoscope (Leica, Germany), or confocal
microscope (Leica SP8, or Olympus Fluoview 1000). Surgical procedures Virus delivery: The surgery area and equipment were sterilized with
70% ethanol, a bead sterilizer and/or autoclaving where possible. Subjects were
anesthetized with 3% isoflurane in an anaesthetic
12 cm 3 chamber. Once fully anesthetized, subjects
were weighed and transferred to a stereotaxic apparatus by gently fixing the
head with ear bars and softly clamping the open snout on a nose piece that
provided continuous isoflurane as anaesthetic blended with oxygen and air to a
minimum of 30% oxygen. Throughout surgery, subjects overlaid a
feedback-controlled heating pad receiving information from a lubricated rectal
probe to assess core temperature (maintained between 35 and 37 °C). Subject
breathing was continually monitored and anaesthesia regulated accordingly. The
subject’s eyes were protected with Vaseline or vitamin A tear gel. Betadine
ointment as aseptic and lidocaine/prilocaine as a topical analgesic (EMLA cream)
were applied topically to the precise incision area on the scalp. An s.c.
injection of Meloxicam (Metacam) analgesic was given in sterile saline
(0.5 mg ml −1 ;
5 µl g −1 ) using a 30G needle. After testing for
analgesia by gentle tail and/or hind paw pinch, a sharp scalpel was used to
expose the skull. All membranes were pushed aside and the skull surface cleaned
with mild hydrogen peroxide (not exceeding 10%) to remove remaining membranes
and bleach the connective tissue, enabling clear visualization of cranial
reference points. A remote, pedal-driven drill affixed to the stereotaxic
manipulator was next used to create a 400 µm diameter craniotomy at coordinates
−0.6 mm from Lamda, 1.0 mm from midline. A stainless steel 33G infusion cannula
(Plastics One, WV, USA) affixed to the manipulator and connected to a 50 µl
gas-tight syringe (Hamilton, Switzerland) via infusion tubing (Plastics One, WV,
USA) and loaded with AAV packaged with EF1a.DIO.hChR2(H134R)-eYFP.WPRE.hGH (AV-1-20298P; Penn Vector
Core, PA, USA) was then lowered at 20° off the normal axis, 3.6 mm beyond the
brain dura. Infusion of 1.0 µl AAV ensued over the course of 10 min
(0.1 µl min −1 ). An additional 5 min were then
allowed for diffusion before the infusion cannula was gradually removed. Finally, the skin was pulled over the skull and sutured with a sterile curved
needed and non-absorbable sutures. Betadine and EMLA cream were again applied to
the now closed surgery area and the subject was removed from the apparatus,
weighed and placed in a clean and heated recovery chamber with close monitoring
until behaving normally. The subjects were then returned to their home cage
(group housed) and monitored at least once a day for 3 days. If any measure from
the postoperative monitoring sheet received a score greater than 1, an
additional dose of general analgesic (Metacam in sterile saline;
0.5 mg ml −1 ; 5 µl g −1 ;
s.c.) was administered. Non-absorbable sutures typically grew out from the skin
within 2 weeks, and if not, were removed during subsequent optical cannula
implant. Optical implants: Implantation of fMRI-friendly optical fibre
cannulae occurred 1–2 weeks post-viral infusion and at least 1 week prior to
ofMRI. Preparation of the surgery area and initial surgery steps proceeded
identically to viral infusions (see ‘virus delivery’ above). Once the skull was
exposed and membranes cleared, a 600 µm hole was drilled into the position for
fibre implantation, directly on midline at Lamda −0.6 mm. A 400 µm optic fibre
extending 3.3 mm beyond the fibre casing obtained from Doric Lenses (Quebec,
Canada) was gently lowered until the casing became flush with the skull. Any
bleeding was cleaned away with the finely-twisted end of a sterile cotton swab. The skull was then re-hydrated by applying PBS with a cotton swap. After
providing about 30 s for the skull to hydrate, a layer of etching reagent (iBond
Total Etch, Heraeus Kulzer, Germany) was applied to the skull using the
manufacturer’s accompanying applicator. After 30 s, another layer of etching
reagent was applied and then fixed with 15 s illumination with a 6 mW blue LED
(Elipar S10, 3M, Switzerland). Optic cannulae were then cemented in place using
light-curing dental cement (Tetric EvoFlow, Ivoclar Vivadent, NY, USA),
providing a minimum of 3 mm of unobstructed cannula above the cement layer to
enable coupling to the optic fibre. Finally, the cannula holder was raised away
from the fibre and the skin fixed to the base of the cement with veterinary
tissue glue (Surgibond, Eisenhut-Vet, Switzerland). Finally, animals were
allowed to recover in an identical manner reported above (see ‘virus
delivery’). Craniotomies for acute electrophysiological recordings in vivo:
Subjects containing optic implants targeting the DRN were anesthetized using 3%
isoflurane in a 30%-minimum oxygen/air blend, and transferred to a mouse
stereotaxic frame providing continuous circulating isoflurane at roughly 2% in
the same gas vehicle mixture as required according to the animal’s breathing. To
provide access of a recording electrode to 5-HT neurons of the DRN, dental
cement was progressively removed using a foot-powered drill on the right side of
the optical cannula until the skull was exposed. For subjects in which dual
recordings were to be made, the cement overlaying the projection ROI was also
removed in an identical manner. Craniotomies were performed by removing the
skull overlaying the cortex lateral to the DRN using the drill at low speed to
gently grind off successive layers of a circle encasing the desired region. Once
the skull at the circle’s edge was completely removed, fine tip forceps were
used to lift away the remaining plate of cortex, and the dura was punctured and
removed with the same tool. Finally, anti-coagulate sponge fully-hydrated with
room temperature PBS was added over the exposed brain. Once all craniotomies
were complete, a bolus of medetomidine (0.1 mg kg −1 )
was delivered s.c., and after 5 min, the concentration of isoflurane was reduced
to 0.5% and medetomidine was continuously delivered at
(0.2 mg kg −1 per hour) s.c., in a manner
identical to the ofMRI experiments. Electrophysiology Patch-clamp recordings in vitro: Mice were decapitated under
isoflurane anaesthesia, and the brains removed in ice-cold oxygenated cutting
solution, containing (in mM): N-methyl d-glucamine (135), KCl (1),
CaCl 2 (0.5), MgCl 2 (1.5),
KH 2 PO 4 (1.2), choline
bicarbonate (20), D-glucose (10), with pH adjusted to 7.4 with HCl (resulting in
a final [Cl-] of ~145 mM). Coronal slices (350 μm) were prepared using a
Vibratome VT1200S (Leica, Germany), transferred to an interface recovery chamber
filled with artificial cerebrospinal fluid (aCSF) containing (in mM): 126 NaCl,
3 KCl, 1.25 NaH 2 PO 4 , 1.2
MgSO 4 , 1 CaCl 2 , 26
NaHCO 3 and 10 glucose, with pH 7.2–7.4 when bubbled
with carbogen gas (95% O 2 and 5%
CO 2 ). The slices were maintained at 32–34 °C for at
least 30 min, before being allowed to cool to room temperature. For recordings,
slices were transferred to a submerged chamber, and superfused with carbogenated
aCSF heated to 32–34 °C at 2–4 ml min −1 . Neurons were
visualized under infrared oblique illumination (Olympus, BX51WI, 40×
water-immersion objective). Whole-cell current-clamp recordings were performed
with glass pipettes (5–8 MΩ), pulled from standard borosilicate glass, and
filled with a pipette solution containing (in mM): 110 potassium-gluconate, 40
HEPES, 2 ATP-Mg, 0.3 GTP, 4 NaCl and 4% biocytin (wt/vol) (pH 7.2–7.3;
osmolarity 280–290 mosmol l −1 ). Recordings were
acquired using a Multiclamp 700B amplifier (Molecular Devices), and digitised
using an ITC-18 A/D board (Instrutech). Blue light was delivered via a
galvanometer-based movable spot illumination system coupled to the
epifluorecscence port of the microscope using a single mode fibre (473 nm,
5–25 ms, UGA-40, Rapp OptoElectronic). Stimulation and recordings were
controlled via custom-written procedures in Igor Pro (Wavemetrics). Isoflurane
was dissolved in an air-tight container of aCSF using conditions previously
shown to induce a final concentration comparable to 1 MAC for C57Bl/6
mice. Multielectrode recordings and optogenetic activation in vivo:
Recordings were performed using single-shank 16 site silicon probes, with
electrode spacings of 25 µm, 100 µm (Neuronexus Technologies Inc., MI, USA) or
200 µm (Cambridge NeuroTech, UK). Recordings from the dorsal raphe were
performed with 25/100 µm spaced electrodes, with recordings from target
structures performed using 100/200 µm spaced electrodes. Each shank was gently
lowered progressively to the desired coordinates (Supplementary
Table 2 ). Recordings from
multielectrode arrays were performed using Brainware (Tucker Davis Technologies,
Alachua, FL, USA), with traces for detecting multiunit activity band-pass
filtered between 0.3 and 3 kHz and digitised at 25 kHz, and traces for LFP
recordings low-pass filtered at 1.9 kHz, digitised at 25 kHz, and down-sampled
by a factor of 8 for file storage. The source of blue light was a 473 nm laser
(Thorlabs, Germany; selected for ease of transport) used to deliver 4–40 mW of
power (Fig. 1I ). Laser power was
controlled with the bench-top unit, and verified with a light meter (PM 160,
Thorlabs, Germany). Pulse duration, inter-stimulus and inter-train intervals
were controlled with in-house software designed in LabView (National
Instruments, Switzerland). At the end of the recording session, the animal was
overdosed with sodium pentobarbitone and perfused with 10–15 ml ice-cold PBS
followed by 10–15 ml ice-cold 4% PFA in PBS. Analysis of electrophysiological data: Data were analysed using
custom-written procedures in Igor Pro (Wavemetrics). Extracellular spikes were
detected as signals exceeding 5 standard deviations of the noise. For recordings
from the dorsal raphe using 25 µm spaced linear probes, an adapted spike sorting
procedure [32] was used to explore whether neurons
displaying specific spike waveforms were selectively recruited by optogenetic
stimulation. Briefly, spike metrics were converted into z scores, over-clustered using an in-built k means algorithm, and progressively aggregated if
the intercluster distance was <2.5 and merging did not produce
violations of refractory period of 2 ms. Analysis was first performed for spikes
which could be observed on 2 channels (stereotrode data), and subsequently on
the residual single channel spikes, with auto-correlation and cross-correlation
plots used to validate the clustering procedure. As several waveform clusters
appeared to exhibit rapid adaptation during optical trains, clusters containing
>50 spikes were included for subsequent analysis. Spike metrics from the
average waveform for each cluster were used to identify different waveform types
via a k means algorithm. This clustering
procedure is likely to be conservative, and underestimate the firing rate of
individual neurons, but was deemed sufficiently robust to detect any bias in
optogenetic recruitment. Significant differences in spiking behaviour were examined with a
Kruskal–Wallis test followed by Dunn’s post-hoc comparison test. Statistics are
reported for combined analysis of stereo and single channel clusters, but the
same pattern of statistical significance was also observed for stereo clusters
alone. Functional magnetic resonance imaging Animal preparation: Animals were anesthetized with isoflurane
(induction 3%, preparation 2%) in a 20/80% O 2 /air
mixture. Animals were positioned on a MRI-compatible cradle equipped with a face
mask, rectal thermometer and adjustable warm water flowing within the support. Animal temperature was kept at 36.5  ± 0.5 °C throughout the experiment. A
cannulae was placed in the tail vein to administer agents. A s.c. line was
placed on the animal flank to administer complementary anaesthetic (Dormitor,
medetomidine hydrochloride; Pfizer Pharmaceuticals, UK). After animal
positioning, a bolus of medetomidine was injected s.c. at
0.1 mg kg −1 . After 5 min post-bolus, isoflurane
was reduced to 0.5% at the initiation of continuous infusion of medetomidine was
initiated (0.2 mg kg −1 per hour) to maintain the
sedation for the remainder of the scanning session. For CBV fMRI experiments,
the paramagnetic iron oxide nanoparticle-based intravascular contrast agent
Endorem® (Laboratoire Guerbet SA, France) was injected at a dose of
30 mg kg −1 Fe, and given 10 min to reach
steady-state prior to imaging. MRI: Functional MRI was performed on a 7 T Pharmascan scanner
(Bruker BioSpin MRI, Ettlingen, Germany), operating at 300 MHz. A custom-built
transmit-receive surface coil was positioned on the head of the animal. A light
fibre connected to a laser (LuxX® 488-60, Omicron, Germany) was positioned
through the coil and attached to the zirconia fibre insert on the mouse head
with a zirconia sleeve. Images acquisition was performed with Paravision 6
software. High-resolution anatomical images were acquired using a gradient echo
FLASH sequence to serve as references with repetition time (TR) 1500 ms, echo
time (TE) 1.97 ms, flip angle (FA) 50°, matrix size (MS) 120 × 120, field of
view 20 × 17.5 mm, slice thickness 0.5 mm, slice gap 0.15 mm, 14 slices. CBV
fMRI was acquired with multi-shot gradient echo EPI using the same geometry as
the anatomical image, 2 segments, TR 1000 ms. TE 5.6 ms, FA 90°, MS 64 × 64,
bandwidth 250,000 Hz, 360 or 720 repetitions for a total duration of 12 and
24 min, corresponding to the short-block (Fig. 2a ) and long-block protocol, respectively. The echo time was
changed to 15 ms for BOLD fMRI. Correction for magnetic field inhomogeneity was
performed with Mapshim using an ellipsoid ROI covering the whole brain. A
trigger device was used to control laser onset with respect to the fMRI scan. Laser power was controlled via the accompanying Omicron software. Laser
stimulation was performed with 6 blocks of 20 s ON and 40 s OFF for 12 min scans
(short-block protocol), and 20 s ON and 160 s OFF for 24 min scans (long-block
protocol), and controlled via an in-house LabView program (National Instruments,
Switzerland). Conditions: Short CBV scans (12 min) were performed in a series of
3 per session: (a) 3 scans with laser power set at 100%, used as a control group
for the subsequent analysis, (b) 3 scans with laser power set at 100%, 66% and
33% in varying order, (c) 1 baseline scan, i.v. administration of Fluoxetine
(4.5 mg kg −1 [29] ), 2
scans post Fluoxetine, (d) 60 min pre-scan animal restrain, 3 scans post
restrain. Data processing: Data processing was performed with FSL (5.0.8, https://fsl.fmrib.ox.ac.uk/ ) and AFNI (2011_12_21_1014, https://afni.nimh.nih.gov/ ) and BROCCOLI (2015-09-11, https://github.com/wanderine/BROCCOLI ) [33] . Anatomical images from each scan session
were linearly aligned with one another, flipped and merged to generate a
symmetrical reference template. Linear and non-linear transformations were
estimated between the anatomical images and the reference template using FLIRT
and FNIRT. Functional images were temporally realigned (3dVolreg), the linear
and non-linear transformations from the anatomical images were then applied to
the functional images. The temporal signal for each region was extracted from a
set of ROIs based on the reference anatomical images. The time series were
linearly detrended to account for the iron nanoparticle clearance, normalised as
percent change to baseline, and the sign inverted. For voxel-wise analysis, the
functional images were smoothed with a 0.45 mm 2 kernel (3dBlurtoFWHM). A GLM first-level analysis was applied to each scan
individually using BROCCOLI. The parameters of the response to the stimulation
blocks were modelled into separate regressors using the default hemodynamic
response function convolution together with temporal derivatives for the
activity regressors and polynomial detrending regressors to account for linear
and non-linear drifts. A contrast was designed to obtain COPE at every voxel. Visual inspection of the residuals from the analysis for each scan suggested the
model accounted fully for the response in the time series for each
condition. Statistical analysis: Second-level between-group voxel-wise
statistics was carried using non-parametric permutation testing implemented in
BROCCOLI. A design matrix modelling scan order for each condition (control,
fluoxetine and restraint) and gender as a covariate was used for the analysis. Fluoxetine versus control comparisons were tested by using a within-session
correction to account for the inter-animal variability. Contrasts were designed
so that the two scans post-drug injection were averaged, and subtracted with the
pre-drug scan and compared against the control scans processed similarly. For
the restrain versus control comparison, within-session correction could not be
applied; all 3 scans in the sessions were averaged and compared against the
control scans. The null distributions for each comparison were estimated using
5000 permutations, and the estimated p -values
were corrected using cluster extend correction. Corrected t -statistic maps are shown as overlay on the AMBMC
template (Australian Mouse Brain Mapping Consortium, https://www.imaging.org.au/AMBMC ). Statistical analysis across ROIs were corrected using false
discovery rate (FDR). Descriptive statistics are given as mean ± 1 standard
deviation. Reporting summary Further information on experimental design is available in
the Nature Research Reporting
Summary linked to this article.